Two-dimensional molybdenum carbide 2D-Mo2C as a superior catalyst for CO2hydrogenation Early transitional metal carbides are promising catalysts for hydrogenation of CO 2 . Here, a two-dimensional (2D) multilayered 2D-Mo 2 C material is prepared from Mo 2 C T x of the MXene family. Surface termination groups T x (O, OH, and F) are reductively de-functionalized in Mo 2 C T x (500 °C, pure H 2 ) avoiding the formation of a 3D carbide structure. CO 2 hydrogenation studies show that the activity and product selectivity (CO, CH 4 , C 2 –C 5 alkanes, methanol, and dimethyl ether) of Mo 2 C T x and 2D-Mo 2 C are controlled by the surface coverage of T x groups that are tunable by the H 2 pretreatment conditions. 2D-Mo 2 C contains no T x groups and outperforms Mo 2 C T x , β-Mo 2 C, or the industrial Cu-ZnO-Al 2 O 3 catalyst in CO 2 hydrogenation (evaluated by CO weight time yield at 430 °C and 1 bar). We show that the lack of surface termination groups drives the selectivity and activity of Mo-terminated carbidic surfaces in CO 2 hydrogenation. Earth-abundant early transitional metal carbides, and in particular carbides of Mo and W, feature catalytic properties similar to those of noble metals [1] , [2] . This property has been exploited for various catalytic processes including Fischer–Tropsch (FT) synthesis [3] , [4] , methane dry reforming [5] , water-gas shift (WGS) reaction [6] , [7] , and CO/CO 2 hydrogenation [8] , [9] . Currently, the conversion of captured CO 2 into value-added chemicals or fuels is considered a key strategy to mitigate the yet increasing anthropogenic CO 2 emissions [10] , [11] , in particular when combined with H 2 obtained using renewable energy [12] , [13] . Depending on the catalyst and the reaction conditions used, thermocatalytic CO 2 hydrogenation can give CO, methanol, dimethyl ether (DME), methane, or heavier hydrocarbons [12] , [14] . In this context, Mo 2 C has been reported as a promising catalyst for CO 2 hydrogenation, yielding a particularly high selectivity to CO via the reverse water-gas shift (RWGS) reaction [8] , [9] , [15] , [16] , [17] . In a recent development, a highly active and selective K-Mo 2 C/γ-Al 2 O 3 catalyst for RWGS has been tested on the pilot scale (ca. 1 kg catalyst) [18] . The activity and selectivity of CO 2 hydrogenation catalysts based on molybdenum carbide can be affected by the C/Mo ratio in the catalyst [19] , [20] . According to density functional theory (DFT) calculations, the Mo-terminated surface of β-Mo 2 C is more reactive for the dissociation of CO 2 than the C-terminated surface [16] , and H 2 dissociation is most favored on the Mo-terminated (001) facet, compared to the C-terminated or mixed Mo/C-terminated facets [21] , [22] . MXenes [23] , [24] , [25] , [26] , [27] , [28] , i.e., a recently discovered family of two-dimensional (2D) early transition metal carbides, nitrides, or carbonitrides with a formula of M n + 1 X n T x ( n = 1, 2, 3, X is C and/or N, and T x are surface oxo, hydroxy, and/or fluoro groups) can be utilized to improve our understanding of the impact of the surface termination groups T x on the catalytic activity and selectivity of metal-terminated carbide surfaces in CO 2 hydrogenation. For instance, delaminated MXene-derived 2D Mo 2 CO x nanosheets dispersed on a silica support were recently shown to feature poor or no activity in the dry reforming of methane if the oxygen coverage is either too low or too high (corresponding to respective Mo oxidation states of ca. +0.2 and +5.5) [29] . Yet the intermediate oxygen coverage of ca. two-thirds of a surface monolayer (Mo oxidation state of ca. +4) provided the highest catalytic activity in DRM, exceeding notably that of bulk β-Mo 2 C. DFT calculations show that the surface termination groups of MXenes affect the adsorption energies of the reaction intermediates by influencing the density of states of the Fermi level [30] . These results and related literature reports illustrate that controlling the surface density and the type of termination groups is an important factor to consider when advancing and deploying carbide-based catalysts [31] , [32] . Multilayered crystalline Mo 2 C T x exhibits a high activity for the WGS reaction [33] . The activity of unreduced Mo 2 C T x is higher relative to Mo 2 C T x that has been partially reduced at 500 °C in 10% H 2 . Interestingly, catalytic tests with 13 C-labeled Mo 2 C T x suggested that carbidic carbon exchanges with 12 CO (reactant gas) and therefore catalysis also proceeds at the interlayer surface of Mo 2 C T x , in addition to the exterior surface. The mentioned reductive defunctionalization of Mo 2 C T x was found to decrease the cell parameter c from ca. 20.51 to ca. 15.63 Å, therefore the lower activity of reduced Mo 2 C T x can be, at least in part, due to increased mass transport limitations into the interlayer space [33] . 2D-Mo 2 C has attracted significant attention for applications as a superconductor [34] , [35] or an electrocatalyst [36] , [37] , however, a robust and scalable synthesis protocol for 2D-Mo 2 C has not been developed yet. Indeed, typical approaches to yield 2D-Mo 2 C exploited so far chemical vapor deposition onto flat substrates and lead to ultra-thin orthorhombic Mo 2 C [38] , [39] . Here, enabled by the scalable synthesis of MXenes [40] , we report a gram-scale synthesis of a phase-pure multilayered hexagonal 2D-Mo 2 C material with only Mo-terminated basal planes. Experimental protocols were developed that allow avoiding the transformation of 2D-Mo 2 C into 3D-Mo 2 C during the reductive removal of T x groups on the Mo 2 C T x surface (Fig. 1a ). Comparing 2D-Mo 2 C and Mo 2 C T x in the catalytic hydrogenation of CO 2 , we find that the coverage of Mo 2 C T x with surface termination groups affects the activity and selectivity appreciably. For instance, abundant T x groups on Mo 2 C T x provide surface acidity, reflected in the formation of DME (among other products) due to the dehydration of methanol; DME is not observed on 2D-Mo 2 C. The latter catalyst features high activity (CO formation rate ca. 6 g h −1 g cat −1 ) for CO 2 hydrogenation and a high selectivity to CO (ca. 94% at 430 °C). 2D-Mo 2 C is by a factor of six per mass of catalyst more active for CO formation at 430 °C than the reference β-Mo 2 C catalyst and shows no deactivation on stream for more than 100 h. Fig. 1: Characterization of Mo 2 C T x and its reduction to 2D-Mo 2 C. a Schematic of the preparation of 2D-Mo 2 C from Mo 2 C T x . b 95 Mo VOCS CPMG MAS NMR spectrum of Mo 2 C T x . c Temperature-programmed reduction of Mo 2 C T x in pure H 2 . d Reduction of Mo 2 C T x followed by in situ Raman spectroscopy with a final isothermal heating step at 500 °C performed for 2 h (see Supplementary Fig. 8 for the stacked Raman spectra). e Reduction of Mo 2 C T x followed by in situ XRD (the peaks of β-Mo 2 C are marked by asterisks and the main reflections of Mo 2 C T x are indexed, see Supplementary Fig. 9 for the 3D plot). 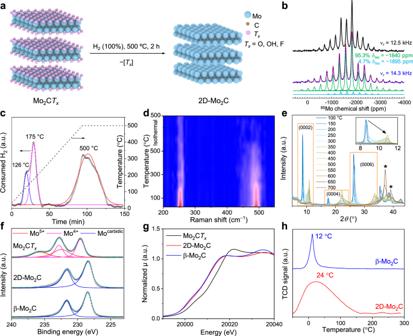Fig. 1: Characterization of Mo2CTxand its reduction to 2D-Mo2C. aSchematic of the preparation of 2D-Mo2C from Mo2CTx.b95Mo VOCS CPMG MAS NMR spectrum of Mo2CTx.cTemperature-programmed reduction of Mo2CTxin pure H2.dReduction of Mo2CTxfollowed by in situ Raman spectroscopy with a final isothermal heating step at 500 °C performed for 2 h (see Supplementary Fig.8for the stacked Raman spectra).eReduction of Mo2CTxfollowed by in situ XRD (the peaks of β-Mo2C are marked by asterisks and the main reflections of Mo2CTxare indexed, see Supplementary Fig.9for the 3D plot).fMo 3dXPS spectra (see Supplementary Table1for the fitting parameters).gMo K-edge XANES spectra of Mo2CTx, 2D-Mo2C, and reference β-Mo2C.hCO temperature-programmed desorption (TPD) of 2D-Mo2C and β-Mo2C. f Mo 3 d XPS spectra (see Supplementary Table 1 for the fitting parameters). g Mo K-edge XANES spectra of Mo 2 C T x , 2D-Mo 2 C, and reference β-Mo 2 C. h CO temperature-programmed desorption (TPD) of 2D-Mo 2 C and β-Mo 2 C. Full size image Synthesis and characterization Multilayered Mo 2 C T x was prepared by Ga etching from Mo 2 Ga 2 C in aqueous HF [33] , [41] . The layered structure of Mo 2 C T x was confirmed by XRD analysis (parameter c = 20.636(3) Å, Supplementary Fig. 1 ), consistent with the lack of a Ga signal in the XPS spectra of Mo 2 C T x (Supplementary Fig. 2 ) [33] , [42] . Raman spectra indicate that the peak due to A 1g ( ω 6 ) Mo−Ga vibrations found at 314 cm −1 in Mo 2 Ga 2 C [43] shifts to 253 cm −1 in Mo 2 C T x , and a new peak emerges at 490 cm −1 due to the surface termination groups (Supplementary Fig. 3 ) [44] . Temperature-programmed oxidation (TPO), performed in a thermogravimetric analyzer, shows that Mo constitutes ca. 73 mass% of Mo 2 C T x (material dried at 80 °C for 24 h), considering that Mo 2 C T x is oxidized to MoO 3 at 600 °C under airflow (Supplementary Fig. 4 ; formation of MoO 3 was confirmed by XRD, see Supplementary Fig. 5 ). The 95 Mo VOCS CPMG MAS NMR spectrum of Mo 2 C T x recorded at 20.0 T shows a set of intense and sharp spinning sidebands arising from a combination of chemical shift anisotropy and quadrupolar interaction. Fitting this spectrum with a single component does not provide a satisfactory result for each individual sideband and therefore a second component is needed. A fit that accounts for all spinning sidebands features a major component centered at −1840 ppm accounting for 95.3% of the full intensity, and a second minor component (4.7%) centered at −1895 ppm. Those positions are slightly dependent on temperature but do not change upon lowering the spinning speed and are hence the isotropic chemical shifts of two distinct molybdenum environments. Those two contributions are displayed in green and light blue respectively, with the experimental spectrum in dark blue and the total simulation in red (Fig. 1b ). It is likely that the major Mo site centered at −1840 ppm corresponds to terrace Mo sites. The structural assignment of the minor site is currently unclear. Yet we cannot exclude that the minor site is due to the edge Mo atoms of Mo 2 C T x nanosheets. We have compared the temperature-programmed reduction (TPR) of Mo 2 C T x in 5% H 2 /Ar and in pure H 2 (50 ml min −1 , ramp 5 °C min −1 ). Mo 2 C T x was heated from 50 to 500 °C, with the off-gas analyzed using a thermal conductivity detector (TCD). We limited the study by 500 °C because of the reported MXene thermal stability limit of ca. 550−600 °C, beyond which the formation of 3D-Mo 2 C occurs [33] . Previous results indicated that the reduction of Mo 2 C T x in dilute H 2 (up to 20%) defunctionalizes T x groups only partially [33] . Three H 2 consumption peaks, at 179, 280, and 500 °C, are identified using 5% H 2 /Ar (Supplementary Fig. 6 ). The low-temperature peak is close to the temperature at which most of the interlayer water desorbs (ca. 179 °C), according to the data of a thermogravimetric differential scanning calorimetry (TGA-DSC) measurement (Supplementary Fig. 7 ), and also consistent with TGA-MS results of Mo 2 C T x in a He atmosphere [45] . The reduction steps at 280 °C likely are associated with the reductive defunctionalization of the surface hydroxyl groups and possibly, fluorine groups, while the peak at 500 °C is related to the removal of surface fluoro and oxo groups [33] , [45] , [46] . When using pure H 2 , the reduction peaks are observed at lower temperatures of 126 and 175 °C, and the peak at 500 °C is significantly more intense as compared to when using 5% H 2 (Fig. 1c and Supplementary Fig. 6 ). This result indicates that the extent of defunctionalization of T x groups at 500 °C can be controlled by the H 2 concentration. An in situ Raman study of the heating of Mo 2 C T x from room temperature to 500 °C under an H 2 flow (100% H 2 , 50 ml min −1 , 5 °C min −1 ), shows that the intensity of the A 1g peak at 253 cm −1 is decreasing with temperature. Interestingly, the E 2g peak at 490 cm −1 (due to T x groups) [44] disappears during the isothermal heat treatment at 500 °C, consistent with the complete removal of the T x groups at this temperature (Fig. 1d and Supplementary Fig. 8 ). Note that the E 2g peak is preserved during the in situ Raman study under Ar [44] , indicating that H 2 plays a critical role in removing the T x groups. The in situ reduction of Mo 2 C T x followed by X-ray powder diffraction (XRD, 5% H 2 /N 2 , 200 ml min −1 , 5 °C min −1 ) shows that the (0002) peak due to Mo 2 C T x (8.5° in the as-synthesized material) shifts, at 500 °C, to a higher angle (10.9°, Fig. 1e ). This change reflects a decrease in the c lattice parameter from 20.64 to 16.21 Å due to the defunctionalization of the T x groups and the removal of intercalated water [33] . The intensity of the (0002) peak decreases starting from ca. 300 °C and increases again at ca. 500 °C, explained by the reestablishing of a long-range order at 500 °C. Compared to Mo 2 C T x reduced in 5% H 2 /N 2 , the material reduced in 100% H 2 (500 °C, 2 h, vide infra, exposed to air prior to the XRD measurement) shows a smaller c parameter of 15.43 Å (the interlayer distance can be roughly estimated as ca. 5 Å), with the (0002) peak shifting to 11.5°. Moreover, the (0004) to (0002) intensity ratio of Mo 2 C T x becomes higher when reduced in 100% H 2 at 500 °C (Supplementary Fig. 10 ), which is related to a change of the coordinates of the Mo atoms [33] . Because of the presence of a crystalline 2D multilayered structure in this reduced material, and the evidence of the complete defunctionalization of the T x groups, as discussed in detail below, we refer to this material hereafter as 2D-Mo 2 C. Increasing the reduction temperature further, the intensity of the (0002) peak decreases and vanishes at 700 °C, implying the loss of the two-dimensional multilayered structure. The diffractogram of Mo 2 C T x -700 matches that of the bulk β-Mo 2 C reference (Supplementary Fig. 10 ). Next, the reductive defunctionalization of Mo 2 C T x was performed in a flow reactor using undiluted H 2 at 500 °C (contact time 0.1 s g cat mL −1 , a total of 2 h) and the resulted 2D-Mo 2 C product was analyzed by X-ray photoelectron spectroscopy (XPS) using an air-tight transfer cell. We observe that the thus obtained 2D-Mo 2 C contains only carbidic Mo sites (Mo 3 d 5/2 binding energy of 228.4 eV) and its spectrum matches that of the bulk β-Mo 2 C reference (also pre-reduced at 500 °C, Fig. 1f , Supplementary Figs. 12 , 13 , and Supplementary Table 1 ). Note that it was reported previously that the reduction of Mo 2 C T x using diluted H 2 (i.e., 20 vol% H 2 in N 2 ) at 500 °C for 1 h defunctionalizes T x groups only partially, leading to Mo 4+ and carbidic Mo states (Mo 3 d 5/2 binding energies at 229.3 and 228.5 eV, respectively) [33] . While a fluorine signal can be clearly observed in the F 1 s XPS data of Mo 2 C T x , H 2 treatment in 100% H 2 at 500 °C for 2 h decreases the F signal in 2D-Mo 2 C to the noise level, consistent with the deep removal of the F groups (Supplementary Figs. 13 and 14 ). The fitted C 1 s region in 2D-Mo 2 C reveals no C−O and COO features and contains only Mo–C and C–C features (vide infra). The control experiment shows that Mo 2 C T x reduced using 10% H 2 /N 2 and under otherwise identical conditions does not give 2D-Mo 2 C owing to the incomplete defunctionalization of T x groups, according to XPS data (Supplementary Fig. 15 and Supplementary Table 1 ) [33] . Scanning electron microscopy (SEM) reveals a similar multilayered hexagonal microstructure for Mo 2 C T x and 2D-Mo 2 C (average hexagonal radius and thickness are 1.0 and 0.3 µm, respectively); in contrast, β-Mo 2 C shows no hexagonal nanoplatelets (Supplementary Figs. 16 − 19 ). An intense fluorine signal in Mo 2 C T x and the lack of thereof in 2D-Mo 2 C are revealed by scanning transmission electron microscopy (STEM) energy-dispersive X-ray analysis (STEM-EDX) (Supplementary Fig. 20 ). A selected area electron diffraction (SAED) pattern of 2D-Mo 2 C displays the Mo-terminated (0002) plane as the main exposed facet, i.e., 2D-Mo 2 C features an almost completely Mo-terminated surface (Supplementary Fig. 21 ). A similar SAED result is observed for Mo 2 C T x -700 , indicating that sintering of the individual layers and formation of the β-Mo 2 C structure (according to XRD results discussed above) retains the Mo-terminated surface (Supplementary Fig. 22 ). In contrast, SAED of β-Mo 2 C shows (0002) and ( \(11\bar{2}0\) ) facets (Supplementary Fig. 23 ), indicating that both Mo-terminated and C-terminated planes are exposed, consistent with a previous study of β-Mo 2 C [16] . The Mo K-edge X-ray absorption near edge structure (XANES) spectrum of 2D-Mo 2 C is clearly different from that of Mo 2 C T x and similar to that of β-Mo 2 C (edge positions 20001.4, 20011.1, and 20000.8 eV, corresponding to the oxidation state of Mo of +0.5, +3.9, and +0.3, respectively, Fig. 1g and Supplementary Fig. 24 ) [33] , [47] . While oxidation states of Mo in 2D-Mo 2 C and β-Mo 2 C are very close, there are changes in the post white line region, likely owing to the different structures of these two carbides (Fig. 1g ). 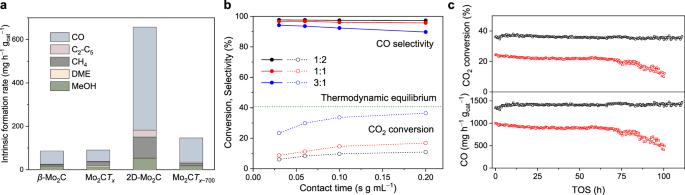Fig. 2: Results of CO2hydrogenation tests. aIntrinsic formation rates obtained after H2pretreatment of Mo2CTxat different temperatures. Reaction conditions: 230 °C, 25 bar, H2/CO2/N2= 3/1/1. Intrinsic formation rates were obtained by extrapolation to zero conversion (zero contact time, see Supplementary Fig.29) and CO2conversion was in the range 0.3−8.5%.bHydrogenation of CO2at 430 °C and 1 bar with 2D-Mo2C under variable H2:CO2ratios. The green dash line shows the calculated thermodynamic equilibrium (based on the minimization of the Gibbs free energy at 430 °C, 1 bar, H2/CO2/N2= 3/1/1).cStability test of 2D-Mo2C (black) and industrial Cu-ZnO-Al2O3(red) at ca. 100 h of TOS (430 °C, 1 bar, H2/CO2/N2= 3/1/1, contact time 0.2 s gcatmL−1). The extended X-ray absorption fine structure (EXAFS) data of β-Mo 2 C can be fitted with a coordination number (CN) to the nearest carbon in the Mo–C shell of 3 and a CN of 6 in the nearest Mo–Mo shell (Supplementary Table 2 and Supplementary Figs. 25 , 26 ). The Mo–Mo shell in 2D-Mo 2 C has a CN of 6.1(7) and a distance of 2.95(1) Å, which are comparable with that of β-Mo 2 C. A CN in Mo–C shell in 2D-Mo 2 C is 2.6(5), i.e., comparable to β-Mo 2 C but significantly lower than in Mo 2 C T x (7(1) for Mo–C/ T x shell). Overall, XANES and EXAFS results are consistent with the formation of 2D-Mo 2 C from Mo 2 C T x . To summarize, all characterization data discussed above suggest 2D-Mo 2 C can be obtained from Mo 2 C T x selectively, i.e., avoiding the formation of 3D-Mo 2 C, if optimized conditions for the complete reductive defunctionalization of T x groups in Mo 2 C T x are used. We performed CO temperature-programmed desorption (TPD) experiments to compare the properties of surface sites in 2D-Mo 2 C, Mo 2 C T x , and the β-Mo 2 C reference. Mo 2 C T x does not absorb CO (Supplementary Fig. 27 ). β-Mo 2 C features a sharp CO desorption peak at 12 °C, indicating uniform Mo sites (Fig. 1h ). In contrast, 2D-Mo 2 C shows a broad CO desorption peak at 24 °C, possibly due to mass transfer effects arising from CO molecules adsorbed also inside the 2D pores of this multilayered material. H 2 TPD results of β-Mo 2 C and 2D-Mo 2 C were also compared. While both materials display well-defined low-temperature desorption peaks centered at −19 and −14 °C for, respectively, β-Mo 2 C and 2D-Mo 2 C, the latter material also has broad H 2 desorption peaks at higher temperatures (ca. 140 and 352 °C) explained by the two-dimensional structure of this carbide and different nature of surface sites in 2D-Mo 2 C (Supplementary Fig. 28 ). Subsequently, CO chemisorption experiments were performed to compare the quantity of exposed Mo sites in the materials under investigation. The CO chemisorption capacity of Mo 2 C T x is very low (0.2 μmol g −1 ), due to abundant surface termination groups (Table 1 ). After H 2 treatment at 300 °C, the amount of chemisorbed CO increases to 14.4 μmol g −1 , indicating the partial removal of the T x groups. 2D-Mo 2 C (prepared in situ prior to CO chemisorption analysis) shows a significantly increased CO capacity of 41.1 μmol g −1 , which exceeds the CO capacity of β-Mo 2 C (also reduced in H 2 at 500 °C in situ) by ca. a factor of eight (Table 1 ). This result is explained by the larger specific surface area of the exposed Mo-terminated facets in 2D-Mo 2 C, which is also consistent with the similar CO 2 adsorption energy of MXenes and 3D transitional metal carbides [48] . H 2 treatment of Mo 2 C T x at 700 °C results in a material with a lower CO capacity (12.8 μmol g −1 ) compared with that of 2D-Mo 2 C due to the sintering of the layered structure of 2D-Mo 2 C, as indicated by XRD, yet the CO capacity is still higher than that of the reference β-Mo 2 C (5.0 μmol g −1 ). Table 1 CO uptake capacities determined by pulse chemisorption measurements. Full size table Catalytic performance The catalytic performance of the prepared materials for CO 2 hydrogenation was evaluated first at 230 °C and 25 bar (H 2 /CO 2 /N 2 = 3/1/1). The main products obtained using Mo 2 C T x are CO, CH 4 , and methanol (intrinsic formation rates of 53, 16, and 13 mg h −1 g cat −1 and intrinsic selectivities of 54, 23, and 11%, respectively) with DME and C 2 –C 5 hydrocarbons as minor products (Fig. 2a and Supplementary Fig. 29 ). The product formation rates are much higher than those from previous studies on the CO 2 reduction by MXene-based electro [49] or photocatalysis [50] . 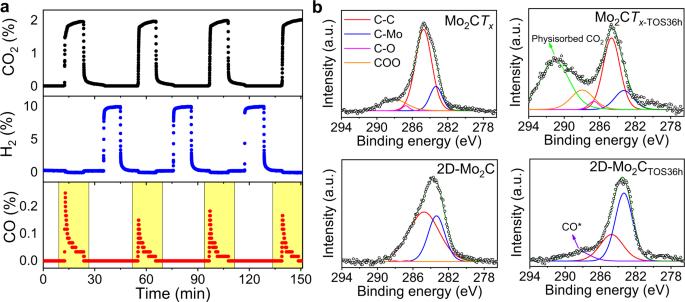Fig. 3: Sequential CO2hydrogenation study. aCO2dissociation study on 2D-Mo2C (430 °C, 1 bar).bC 1sXPS regions of fresh and used Mo2CTxand 2D-Mo2C catalysts, i.e., before and after their exposure to the reaction stream. All intrinsic formation rates and intrinsic selectivities reported in this work (Supplementary Table 3 ) are derived from contact time studies using extrapolation to zero conversion (i.e., zero contact time). The low CO chemisorption capacity of Mo 2 C T x increases significantly after a 1-h exposure to an H 2 /CO 2 mixture (3/1, 1 bar), reaching 4.6 μmol g −1 (Table 1 ). This result indicates that the T x groups in Mo 2 C T x are partially removed under CO 2 hydrogenation conditions. A minor amount of DME (8% selectivity) is formed on Mo 2 C T x ; this product is not observed when using the β-Mo 2 C or 2D-Mo 2 C catalysts (Fig. 2a and Supplementary Fig. 30 ). DME is a typical product of methanol dehydration on Brønsted or strong Lewis acid sites [51] , [52] , [53] , which suggests strong acidity in Mo 2 C T x . Indeed, the NH 3 TPD experiment reveals intense NH 3 desorption peaks at ca. 120 and 500 °C in Mo 2 C T x that had been exposed to an H 2 /CO 2 mixture (3/1, 1 bar) for 1 h (Supplementary Fig. 31 ). Interestingly, while the related MXene material, Ti 3 C 2 T x , has been reported to give no NH 3 desorption peaks, Brønsted and Lewis acidity was found in Ti 3 C 2 T x using pyridine as a probe molecule [54] . Brønsted acidity of highly oxophilic Mo 2 C has been reported previously to appear after the exposure of Mo 2 C to oxygen; in contrast, no significant acidity is observed for reduced β-Mo 2 C [55] , which is also consistent with the NH 3 TPD results of materials of this study, i.e., β-Mo 2 C, 2D-Mo 2 C, and Mo 2 C T x -TOS1h (Supplementary Fig. 31 ). Fig. 2: Results of CO 2 hydrogenation tests. a Intrinsic formation rates obtained after H 2 pretreatment of Mo 2 C T x at different temperatures. Reaction conditions: 230 °C, 25 bar, H 2 /CO 2 /N 2 = 3/1/1. Intrinsic formation rates were obtained by extrapolation to zero conversion (zero contact time, see Supplementary Fig. 29 ) and CO 2 conversion was in the range 0.3−8.5%. b Hydrogenation of CO 2 at 430 °C and 1 bar with 2D-Mo 2 C under variable H 2 :CO 2 ratios. The green dash line shows the calculated thermodynamic equilibrium (based on the minimization of the Gibbs free energy at 430 °C, 1 bar, H 2 /CO 2 /N 2 = 3/1/1). c Stability test of 2D-Mo 2 C (black) and industrial Cu-ZnO-Al 2 O 3 (red) at ca. 100 h of TOS (430 °C, 1 bar, H 2 /CO 2 /N 2 = 3/1/1, contact time 0.2 s g cat mL −1 ). Full size image H 2 pretreatment at 300 °C (100% H 2 , 2 h) does not change appreciably the activity and selectivity of Mo 2 C T x (Supplementary Fig. 29 ). In contrast, H 2 pretreatment at 500 °C (2 h) yields 2D-Mo 2 C and impacts the catalytic performance significantly (Fig. 2a ). In particular, the intrinsic methanol formation rate for 2D-Mo 2 C is 53 mg h −1 g cat −1 , which is comparable to the activity of the Cu-ZnO-ZrO 2 catalyst (37 wt% Cu loading, ca. 45 mg h −1 g cat −1 ) in similar (220 °C, 30 bar, H 2 /CO 2 = 3/1) conditions [56] . The formation rates of CO and C 2 –C 5 hydrocarbons increase as well for 2D-Mo 2 C, reaching 475 and 32 mg h −1 g cat −1 ; these values are ca. 9 and 19 times higher than those obtained using Mo 2 C T x (Supplementary Table 3 ). Thus, the higher activity of 2D-Mo 2 C relative to Mo 2 C T x correlates with the trend in CO chemisorption as discussed above (Table 1 ). Noteworthy, the activity observed for 2D-Mo 2 C is higher than for Mo 2 C T x despite the reduced interlayer distance in 2D-Mo 2 C (unit cell parameters c is 15.43 and 20.64 Å in 2D-Mo 2 C and Mo 2 C T x , respectively; 2D-Mo 2 C was exposed to air prior to the XRD measurement). This result is also different from that found in a recent DRM study, where an oxycarbidic 2D-Mo 2 CO x with an average Mo oxidation state of +4 (modeled by the 2/3 of a monolayer oxygen surface coverage) is the active phase [29] . Interestingly, our previous study showed that Mo 2 C T x is more active in the WGS reaction (CO + H 2 O ↔ CO 2 + H 2 ) than Mo 2 C T x pretreated under 10% H 2 /N 2 at 500 °C for 1 h (i.e., only a partially reduced material) [33] . We have suggested that the reduced interlayer distance of the pretreated catalyst may lead to increased mass transport limitations in the interlayer space [33] . In this study, we have compared the activity of Mo 2 C T x and 2D-Mo 2 C for WGS at 500 °C (CO/H 2 O/N 2 = 1/1/9). Mo 2 C T x shows a stable activity for at least 10 h of TOS, consuming CO at a rate of ca. 5.6 g h −1 g cat −1 (>99% selectivity to CO 2 at 49% conversion of CO). However, while the initial activity of 2D-Mo 2 C is similar to that of Mo 2 C T x (ca. 4.8 g h −1 g cat −1 ), in the first 4 h of TOS it decreases to ca. 2.8 g h −1 g cat −1 of consumed CO (>99% selectivity to CO 2 at 25% conversion of CO, Supplementary Fig. 32 ). XANES data reveals that 2D-Mo 2 C is oxidized under the WGS conditions used, reaching after 10-h of TOS an oxidation state (and therefore a T x surface coverage) close to that of Mo 2 C T x (Supplementary Fig. 33 ). Owing to this similar T x surface coverage, the lower activity of 2D-Mo 2 C after 4-h of TOS is consistent with mass transport limitations due to the reduced interlayer distance in the H 2 -pretreated Mo 2 C T x materials. The decrease of the activity of 2D-Mo 2 C in the first 4 h of TOS is therefore linked with the slow surface oxidation (likely, by steam) of 2D-Mo 2 C, including the interlayer Mo sites. Note that such significant oxidation of 2D-Mo 2 C under WGS conditions contrasts substantially the only minor oxidation of 2D-Mo 2 C in RWGS conditions (vide infra). 2D-Mo 2 C shows a ca. eight times higher intrinsic CO 2 hydrogenation reaction rate normalized per catalyst mass compared to β-Mo 2 C (Supplementary Table 3 ). In other words, the intrinsic rates of CO 2 consumption normalized by surface Mo sites determined by CO chemisorption in 2D-Mo 2 C and β-Mo 2 C are similar. This is in sharp contrast with the significantly higher specific activity of 2D-Mo 2 CO x relative to β-Mo 2 C in the dry reforming of methane [29] . If we compare the intrinsic product formation rates normalized by surface Mo sites, the rate of CO formation is also similar on 2D-Mo 2 C and β-Mo 2 C. These results indicate that the increased activity of 2D-Mo 2 C (per mass catalyst) is mostly due to the greater fraction of exposed Mo atoms available for the catalytic reaction in the 2D material. However, the formation rate normalized by surface Mo of C 1 −C 5 is higher on 2D-Mo 2 C relative to β-Mo 2 C (33 vs. 18 g h −1 g surf(Mo) −1 ), which is offset by the lower methanol formation rate (14 vs. 35 g h −1 g surf(Mo) −1 , Supplementary Fig. 34 ). This difference suggests that other factors are also in play, possibly related to differences in the adsorption energies of reactive intermediates in these two catalysts. We have performed a control experiment and compared the activities of 2D-Mo 2 C and the material obtained after the pretreatment of Mo 2 C T x in 10% H 2 at 500 °C for 2 h. The latter catalyst denoted Mo 2 C T x -500-10% shows lower formation rates of hydrogenation products (Supplementary Fig. 35 ). This inferior activity is explained by the incomplete defunctionalization of T x groups in Mo 2 C T x -500-10% as confirmed by XPS data (Supplementary Fig. 15 ). Furthermore, a reduction of Mo 2 C T x under pure H 2 at 700 °C leads to a notably lower catalytic activity (Fig. 2a ), as compared to 2D-Mo 2 C, explained by the formation of 3D-Mo 2 C (Supplementary Fig. 10 ). This trend is in agreement with the CO chemisorption results (Table 1 ). The catalytic performance of Mo 2 C T x and 2D-Mo 2 C was then compared at three additional temperatures, i.e., 130, 330, and 430 °C at 25 bar using an H 2 :CO 2 ratio of 3. The results show that the distribution of products on Mo 2 C T x and 2D-Mo 2 C depends on the reaction temperature, in agreement with the thermodynamic calculations (Supplementary Figs. 36 − 39 ). More specifically, at 130 °C, a high methanol selectivity of 41 and 62% is observed for Mo 2 C T x and 2D-Mo 2 C, respectively. Increasing the reaction temperature from 130 to 430 °C, increases the intrinsic CO selectivity for Mo 2 C T x from 44 to 91%, yet the CO selectivity for 2D-Mo 2 C increases only from 31% at 130 °C to 65% at 230 °C, before it decreases again to 35 and 39% at 330 °C and 430 °C, respectively. (Supplementary Fig. 39 ). In contrast, the intrinsic selectivity to C 1 −C 5 hydrocarbons increases from 6% at 130 °C to 61% at 430 °C with 2D-Mo 2 C. Among the C 1 −C 5 hydrocarbons, CH 4 is the major component with a partial selectivity of 83% among the C 1 −C 5 products; C 2 −C 5 hydrocarbons are predominantly alkanes (>99%, Supplementary Fig. 40 ). Given the known activity of Mo 2 C-based catalysts in the FT process [3] , the formation of C 2 −C 5 hydrocarbons can be explained by the FT activity of 2D-Mo 2 C with H 2 and CO formed in situ by the hydrogenation of CO 2 . We note that the hydrogenation of propene (formed in situ from propyne) to propane has been reported to occur on molybdenum carbides above 300 °C [57] . Next, contact time studies were also performed at lower pressures, i.e., 1 bar and 5 bar, using 230 °C and an H 2 :CO 2 ratio of 3. At 1 bar, CO is the main product for both Mo 2 C T x and 2D-Mo 2 C (73 and 90% selectivity, respectively), in agreement with thermodynamic calculations (Supplementary Figs. 36 , 41 − 43 ). Increasing the reaction pressure leads to an increase in the formation rates of all products (Supplementary Figs. 41 and 42 ), while the selectivity to CO decreases. The highest selectivity to CO is obtained at a low H 2 :CO 2 ratio of 1:2, and increasing the H 2 :CO 2 ratio increases the selectivities to other products (methanol, DME, and hydrocarbons, see Supplementary Figs. 44 − 46 ). Overall, at all conditions tested, the intrinsic formation rates for the different products are higher on 2D-Mo 2 C relative to Mo 2 C T x except for DME, which is not observed on 2D-Mo 2 C. Based on the above results and those of the thermodynamic calculation (Supplementary Fig. 36 ), we performed a CO 2 hydrogenation test at 430 °C and 1 bar to evaluate the maximized weight time yield (WTY) of CO. In these conditions, the selectivity to CO is high (90−99%) for both Mo 2 C T x and 2D-Mo 2 C, with the selectivities depending on the H 2 :CO 2 ratio tested (1:2, 1:1, 3:1) and the contact time (Fig. 2b and Supplementary Fig. 47 ). A high CO formation rate of ca. 6 g h −1 g cat −1 is obtained with 2D-Mo 2 C at 0.03 s g cat mL −1 contact time and an H 2 :CO 2 ratio of 3:1, i.e., six times higher than obtained with β-Mo 2 C (Supplementary Fig. 48 ). Keeping these conditions the same, but changing the contact time to 0.2 s g cat mL −1 , yields a CO 2 conversion that is close to the thermodynamic equilibrium (Fig. 2b ). This WTY of CO exceeds reported values for the RWGS reaction on Cu-Mo 2 C (Cu loading 1 wt%) at similar reaction conditions [58] or the benchmark Cu-ZnO-Al 2 O 3 (Cu loading ca. 60 wt%) catalyst (Supplementary Fig. 48 ) tested at identical reaction conditions, indicating a remarkable catalytic activity of 2D-Mo 2 C for the RWGS. We also performed a catalytic test of 2D-Mo 2 C at 430 °C and 25 bar. In contrast to β-Mo 2 C or the Cu-ZnO-Al 2 O 3 catalysts, 2D-Mo 2 C can be made selective for methane, i.e., >80% selectivity to methane can be achieved at a long contact time of 2.4 s g cat mL −1 (Supplementary Fig. 49 ). Therefore, 2D-Mo 2 C is a more versatile catalyst for CO 2 hydrogenation compared to the conventional β-Mo 2 C or Cu-ZnO-Al 2 O 3 catalysts. Turning to catalytic stability, the catalytic performance of Mo 2 C T x is stable over 36 h of TOS at 230 °C (25 bar, H 2 /CO 2 /N 2 = 3/1/1, Supplementary Fig. 50 ). However, after 36 h of TOS at a higher temperature of 430 °C (material denoted Mo 2 C T x -TOS36h(430) ), the catalytic activity of Mo 2 C T x changes significantly when the reaction temperature is decreased to 230 °C. The formation rate of CO increases from 62 to 116 mg h –1 g cat –1 , and the formation rate of C 2 –C 5 increases from 4 to 10 mg h –1 g cat –1 . DME is not observed at 230 °C after 36 h of TOS at 430 °C, indicating the loss of acidity of the catalyst. XRD result shows that the c parameter decreases to 15.41 Å (Supplementary Fig. 51 ), indicating that the multilayered material undergoes a reduction in the interlayer spacing. Mo K-edge XANES shows that the Mo white line and the edge position are shifted to lower energies after reaction at 430 °C (Supplementary Fig. 52 ), in agreement with the reduction of Mo. Likewise, Mo 3 d XPS also shows that the material is reduced in situ during the reaction at 430 °C, with the Mo 5+ fraction decreasing from 46 to 31% and the carbidic Mo fraction increasing from 0 to 8% (Supplementary Fig. 53 and Supplementary Table 1 ). This indicates that the activity change of Mo 2 C T x -TOS36h(430) is caused by the reduction of Mo with time on stream. Subjecting Mo 2 C T x -TOS36h(430) to 100% H 2 at 500 °C for 2 h further increases its activity, making it very close to that of 2D-Mo 2 C (Supplementary Fig. 54 ). 2D-Mo 2 C shows no deactivation after more than 100 h TOS at 430 °C (1 bar, H 2 /CO 2 /N 2 = 3/1/1), with a stable CO 2 conversion and CO formation rate. In contrast, the industrial Cu-ZnO-Al 2 O 3 catalyst deactivates in these conditions by ca. 50% (Fig. 2c ), likely due to the oxidation of Cu and/or agglomeration of ZnO. XRD analysis of the used catalyst shows no change of the multilayered structure of the 2D-Mo 2 C (Supplementary Fig. 55 ). Operando Raman study shows that there is no reappearance of a band at 490 cm −1 due to surface termination groups, as was observed in the as-synthesized Mo 2 C T x discussed above (Supplementary Fig. 56 ). However, Mo K-edge XANES data show that the edge position increases from 20001.4 to 20002.0 eV after reaction (Supplementary Fig. 57 ), indicating that Mo becomes slightly more oxidized, i.e., the average oxidation state of Mo in used 2D-Mo 2 C is slightly higher relative to that in fresh 2D-Mo 2 C (Supplementary Fig. 24 ). This is also confirmed by 13 C MAS NMR analysis of the used 2D-Mo 2 C (vide infra). Mechanistic study Decoupling of the oxidation and reduction steps in CO 2 hydrogenation (i.e., operation in a chemical looping scheme) can be beneficial for the separation of products and an improved energy integration due to operation in separate exo/endothermic half reactions [59] . To investigate whether the oxidation and reduction steps can be decoupled for the net CO 2 hydrogenation reaction, we flowed 2% CO 2 in N 2 through a fixed bed of 2D-Mo 2 C (100 mg) at 430 °C and 1 bar and detected that 294 μmol g −1 of CO has been formed in 10 min (Fig. 3a ). After regeneration with 10% H 2 at 430 °C for 10 min, a lower CO amount is detected in the second cycle (176 μmol g −1 , Supplementary Table 4 ), indicating that 2D-Mo 2 C cannot be fully recovered in 10% H 2 . No further deactivation is observed from the second to the fourth cycle. A similar catalytic test was then performed in a TGA, where the reduction and oxidation of the catalyst could be monitored by the mass change (Supplementary Fig. 58 ). The sample mass after the second H 2 treatment is 0.5 wt% higher compared to that after the original H 2 reduction, providing further evidence for the partial oxidation of Mo (formation of 2D-Mo 2 CO x ) with TOS, as also suggested by the Mo K-edge XAS data. In sharp contrast, the amounts of CO formed under identical chemical looping conditions but using β-Mo 2 C was below the detection limit of the infrared detector (Supplementary Fig. 59 ). While these chemical looping type experiments demonstrate that H 2 is not required to be involved in the CO formation step from CO 2 on 2D-Mo 2 C, we cannot exclude that CO formation under RWGS conditions involves formate intermediates [60] . Fig. 3: Sequential CO 2 hydrogenation study. a CO 2 dissociation study on 2D-Mo 2 C (430 °C, 1 bar). b C 1 s XPS regions of fresh and used Mo 2 C T x and 2D-Mo 2 C catalysts, i.e., before and after their exposure to the reaction stream. Full size image 13 C MAS NMR data of the used (and still active) 2D-Mo 2 C catalyst after 9 h of TOS (430 °C, 1 bar, H 2 /CO 2 /N 2 = 3/1/1) was recorded (Supplementary Fig. 60 ). The decreased intensity of the carbon peak at 175 ppm (oxycarbide carbon) and the appearance of a new broad peak at 275 ppm (carbidic carbon) confirms that 2D-Mo 2 C is oxidized slightly under the reaction conditions [33] , [61] . However, the broad peak at 275 ppm may also contain a contribution from surface C* species. The 95 Mo NMR spectrum of the used 2D-Mo 2 C catalyst was difficult to obtain since the compound did not spin in a 20.0 T magnetic field; this behavior is characteristic for materials with metallic conductivity. Recording the spectrum under static conditions yields a very broad spectrum spanning almost 5000 ppm (Supplementary Fig. 61 ). This observation is fully consistent with the very broad line observed for a Mo/ZSM-5 catalyst at an ultra-high field and is assigned to Mo 2 C/MoO x C y species [62] . A fit of the spectrum (neglecting Knight shifts) estimates the isotropic chemical shift at 615 ± 100 ppm, in good agreement with the 900 ppm value found for Mo 2 C [63] . We observe a quadrupolar coupling constant C Q of ca. 20.6 ± 0.1 MHz, which is much larger than the C Q of 6.1 MHz found for Mo 2 C. In addition, we find in our used 2D-Mo 2 C catalyst that a quadrupolar asymmetry parameter η Q = 0.0 ± 0.15, as opposed to η Q = 0.98 that is found in Mo 2 C. This low η Q value is consistent with a cylindrical symmetry of the Mo environment in low-dimensional Mo sites (i.e., 2D-morphology) in used 2D-Mo 2 C. To assess the nature of carbonaceous surface species in working catalysts, we compared the C 1 s XPS data of Mo 2 C T x and 2D-Mo 2 C catalysts before and after their exposure to the reaction stream at 430 °C, 1 bar, 36 h (Fig. 3b and Supplementary Figs. 62 , 63 ). CO 2 physisorbed on Mo 2 C T x is identified by a peak with a binding energy of ca. 291.0 eV [8] . As such peak is not observed on 2D-Mo 2 C it is suggested that CO 2 is converted rapidly on the surface of 2D-Mo 2 C under reaction conditions; instead, surface CO species (low intensity feature with a fitted maximum position at 288.9 eV) are observed on 2D-Mo 2 C after exposure to the reaction stream. To conclude, we have shown that the activity and selectivity of multilayered Mo 2 C T x catalysts under CO 2 hydrogenation conditions can be tuned by controlling the surface termination groups through H 2 treatment. A T x -free, Mo-terminated 2D-Mo 2 C is synthesized by treatment in pure H 2 at 500 °C. 2D-Mo 2 C is more active for the RWGS reaction compared to β-Mo 2 C and the Cu-ZnO-Al 2 O 3 reference. With the CO yield close to the thermodynamic equilibrium at 430 °C (that is in harsh, H 2 O-reach conditions), the 2D-Mo 2 C is stable for more than 100 h TOS under the studied reaction conditions. As the exposed terrace surface of 2D-Mo 2 C is purely Mo-terminated, its CO chemisorption capacity exceeds that of β-Mo 2 C by a factor of ca. eight, leading in turn to a comparable increase of its activity in the hydrogenation of CO 2 to CO. 2D-Mo 2 C is highly active for CO 2 dissociation and can also be used in the chemical looping CO 2 -H 2 redox cycles. Overall, the results obtained indicate that 2D-Mo 2 C is a promising catalyst for CO 2 hydrogenation, exhibiting a remarkable catalytic activity and stability. Material synthesis Mo 2 Ga 2 C was synthesized following a previously reported method [33] , [64] , [65] . β-Mo 2 C (1 g, Sigma-Aldrich, 99.5 wt%) was mixed with metallic gallium (3 g, Alfa Aesar, 99.99 wt%) at 45 °C to obtain a mirror-like paste. The paste was flame-sealed under dynamic vacuum (ca. 10 −5 mbar) and annealed at 850 °C for 48 h. The solid was then stirred in 12 M HCl (20 mL, VWR Chemicals) at room temperature for 48 h and washed with water until a pH of ca. 6 was reached. The powder was then dried at 80 °C overnight to obtain Mo 2 Ga 2 C. Mo 2 C T x was prepared by stirring Mo 2 Ga 2 C (1 g) in 50 mL of HF solution (14 M, Sigma-Aldrich) at 400 rpm in a sealed Teflon-lined autoclave for 10 days at 140 °C [33] . It should be noted that experiments with highly toxic concentrated HF solutions should be conducted in a dedicated fume hood and require extra care. After washing with deionized water until a pH of ca. 6 is reached and drying at 80 °C overnight the Mo 2 C T x powder was obtained. Mo 2 C T x –300 and 2D-Mo 2 C were prepared by treating the Mo 2 C T x at 300 and 500 °C for 2 h (heating rate 5 °C min −1 ) under 100% H 2 , respectively. The industrial CuO-ZnO-Al 2 O 3 catalyst (63.5 wt% CuO, 25 wt% ZnO, 10 wt% Al 2 O 3 , and 1.5 wt% MgO fume) was obtained from Alfa Aesar and reduced at 500 °C before the catalytic test. All the materials were kept in a glovebox prior to characterization and catalytic tests. Except for XRD, ex situ characterization data of the activated materials have been acquired in pristine conditions, i.e., without exposure to air. Material characterization Powder X-ray diffraction (XRD) data were collected on a PANalytical Empyrean X-ray diffractometer with a Bragg-Brentano HD mirror operated at 45 kV and 40 mA using Cu K α radiation ( λ = 1.5418 Å). The materials were scanned in the 2 θ range of 5–90° using the step size of 0.0167° and a scan time per step of 3 s. In situ XRD was performed in the same instrument using an Anton Paar XRK 900 reactor chamber, in the range of 5–45° from room temperature to 700 °C (5 °C min −1 ) under 5% H 2 /Ar. XPS was performed on a Sigma 2 instrument (Thermo Fisher Scientific) with a UHV chamber (nonmonochromatic 200 W Al K α source, a hemispherical analyzer, and a seven-channel electron multiplier). The analyzer-to-source angle was 50° and the emission angle was 0°. An air-tight cell was used to transfer samples (supported on carbon tapes) from the glovebox to the XPS chamber without exposure to air [66] . The X-ray absorption spectra at the Mo K-edge were measured at the SuperXAS beamline at the Swiss Light Source (Paul Scherrer Institute, Villigen, Switzerland), operating in top-up mode at 2.4-GeV electron energy and a current of 400 mA. XAS data were collected at the Mo K-edge using a Si (111) monochromator in transmission mode between 19,800 and 21,150 eV with a step size of 0.25 eV. The calibration of the XAS data was based on the Mo foil at 20,000 eV. The sample was pressed into a pellet with an optimized amount of sample mixed with cellulose and sealed in air-tight aluminized plastic bags in the glovebox. The processing of the XAS data was performed with ProQEXAFS and Athena software [67] , [68] . The EXAFS fitting was conducted with the Artemis software [68] . The fitted variables include the CN, interatomic distance R , bond length disorder factors (Debye–Waller factors, DW), and energy shift. The amplitude reduction factor S 0 2 = 0.96 was obtained from fitting the corresponding Mo foil. Data fitting was carried out in the range of 1.0−3.0 Å and with a window Δ R of 0.5; the Fourier transform was carried out for k = 3.0−15.0 Å −1 . TEM measurements were performed on an FEI Talos F200X transmission electron microscope operated at 200 kV. The STEM measurements were carried out in the same instrument with a resolution of 0.16 nm and a high-angle annular dark-field (HAADF) detector. The energy-dispersive X-ray spectroscopy (EDX) was obtained with a Super-X EDS system (windowless, shutter protected). SEM measurements were conducted on an FEI Magellan 400 FEG microscope (0.05–30 kV) with an EDAX Octane Elect Super EDS System. Before the measurement, the sample was sputter-coated with a ca. 5 nm layer of PtPd. H 2 TPR, NH 3 TPD, CO TPD, H 2 TPD, and CO chemisorption were performed on an AutoChem (Micromeritics) instrument with a TCD. Ca. 100 mg of the specimen was loaded in a U-shape quartz reactor. The H 2 TPR was performed under 5% H 2 /Ar from room temperature to 500 °C with a heating rate of 10 °C min –1 . In a typical NH 3 TPD experiment, the sample was pretreated at 300, 500, or 700 °C under pure H 2 for 2 h, saturated in 5% NH 3 /He flow for 30 min at 50 °C, and purged with He for another 30 min. After that, the sample was heated to 1000 °C at 10 °C min −1 under He flow and the desorbed NH 3 was monitored with the TCD detector. A similar experiment without NH 3 introduction was conducted to obtain the background. CO TPD and H 2 TPD were performed following similar procedures from −50 °C. For CO chemisorption, the sample was first pretreated at 300, 500, or 700 °C under pure H 2 for 2 h, and the CO adsorption isotherm were acquired at 0 °C. The TGA-TPR study was performed in a Mettler Toledo TGA-DSC 3+ under 10% H 2 /N 2 from room temperature to 500 °C at the heating rate of 5 °C min −1 . The temperature-programmed oxidization (TPO) study in a TGA was performed under air from room temperature to 800 °C using a heating rate of 5 °C min −1 . Raman spectroscopy was performed in a DXR 2 Raman spectrometer (Thermo Fisher) using a 532 nm excitation laser. During the measurement, the sample was loaded in an in situ cell (Linkam CCR1000) with flowing N 2 to protect the sample from damage by the laser. For the operando Raman study, the sample was first pretreated in pure H 2 at 500 °C for 2 h, followed by flow H 2 /CO 2 /N 2 (3/1/1) under 1 bar at 430 °C for 2.5 h. The 95 Mo solid-state NMR spectra were obtained at a principal magnetic field of 20.0 T (i.e., a Larmor frequency of 55.1 MHz) using a 4 mm diameter rotor, spinning at 14.3 kHz, and with a temperature set at 5 °C. The radio-frequency field used was 25 kHz, leading to an optimum 90° pulse of 5.0 µs and a CPMG sequence summing 30 echos was able to significantly increase the signal-to-noise ratio. Under those conditions, a Hahn Echo sequence did not provide a sufficiently large irradiation bandwidth to fully cover the extent of the spectra and we applied a VOCS procedure [69] , [70] , recording 11 spectra separated by a 50 kHz offset. In total, 16k scans were acquired with a recycle delay of 0.5 s for each sub-spectrum. The spectra are referenced to a 2 M solution of Na 2 MoO 4 . Further details are provided in the Supplementary Information file. Catalytic testing The CO 2 hydrogenation reactions were conducted in a high-pressure tubular reactor (304.8 mm of length, 9.1 mm of internal diameter, Hastelloy X, Microactivity Effi, PID Eng&Tech) as reported in our previous study [71] . For a typical reaction, the catalyst (50 mg) was loaded in the glovebox and transferred without exposure to air. The H 2 treated catalysts Mo 2 C T x -300 and 2D-Mo 2 C were prepared in situ prior to the catalytic tests under an H 2 flow (50 mL min –1 , 10 °C min –1 , 2 h). Before the reaction, the catalyst was protected under N 2 to the designated temperature (10 °C min –1 , 130–430 °C) and charged to the designated pressure (1–25 bar) with N 2 . The gas feed was then switched to the reaction gas mixture of H 2 , CO 2 , and N 2 with a specific H 2 /CO 2 ratio (1/2, 1/1, or 3/1) and 20 vol% N 2 as a balance. The products were analyzed online by double-channel gas chromatography (PerkinElmer Clarus 580) with the transfer line heated to 150 °C. H 2 , N 2 , and CO 2 were analyzed in Channel A equipped with a RESTEK ShinCarbon ST Micropacked Column and a TCD. CO, CH 4 , methanol, DME, and C 2 –C 5 hydrocarbons were analyzed in Channel B with an Agilent HP-PLOT Q Column, a methanizer, and a flame ionization detector. Different contact times (space velocities) were probed by changing the gas flow rate from 100 to 15 NmL min –1 . The product formation rate, CO 2 conversion, and selectivity to the given product were calculated with the following equations: 
    F_x,out[mol h^-1]=C_x,out× F_N_2,in/C_N_2,out
 (1) 
    r_x[g h^-1g_cat^-1]=F_x,out/m_cat×MW_x
 (2) 
    X_CO_2=∑_i=1^nF_x,out/F_CO_2,in
 (3) 
    S_x=F_x,out/∑_i=1^nF_x,out
 (4) where F x, out is the outlet flow rate of species x [mol h −1 ]; C x, out is the outlet gas fraction of species x ; F x, in is the inlet flow rate of species x [mol h −1 ]; r x is the formation rate of species x [g h −1 g cat −1 ]; m cat is the mass of catalyst used in the reaction [g]; MW x is the molecular weight of species x [g mol −1 ]; X CO2 is the conversion of CO 2 ; S x is the selectivity of species x . Intrinsic formation rates were extrapolated using a second-order polynomial fit to the experimental data. Intrinsic selectivities were calculated from the intrinsic formation rates. The WGS reaction was performed in a fixed-bed quartz reactor (400 mm of length and 12.6 mm of internal diameter) at atmospheric pressure. Mo 2 C T x (30 mg) was supported on a plug of glass wool and the 2D-Mo 2 C catalyst was prepared in situ prior to the catalytic test. The WGS reaction was performed under a stream of CO, H 2 O, and N 2 (total flow rate 55 mL min −1 , CO/H 2 O/N 2 = 1/1/9) at 500 °C for 10 h. The steam was generated from water evaporation with an evaporation mixer (Bronkhorst) and the water flow rate was controlled by a liquid flow meter (Bronkhorst, μ-Flow series). The off-gas after condensation of the unreacted steam was analyzed by double-channel gas chromatography (PerkinElmer Clarus 580) with thermal conductivity and flame ionization detectors. The CO 2 dissociation experiments were performed in a tubular reactor. At 430 °C, the catalysts were exposed to 2% CO 2 /N 2 (100 mL min −1 ) for 10 min, purged with N 2 (100 mL min −1 ) for 10 min, and reactivated with 10% H 2 /N 2 (100 mL min −1 ). The gases were measured online using a gas analyzer (ABB, EL3020) with a frequency of 1 Hz. A similar experiment was performed in a TGA (Mettler Toledo). Here, ca. 50 mg of Mo 2 C T x was loaded in a sapphire crucible and treated in 10% H 2 /N 2 (100 mL min −1 ) at 500 °C for 2 h (10 °C min −1 ). The sample was then cooled to 430 °C in N 2 and treated with 10% CO 2 /N 2 for 6 h. After purging with N 2 for 10 min, the sample was treated with 10% H 2 /N 2 (100 mL min −1 ) for another 6 h. Three cycles were performed between 10% CO 2 /N 2 and 10% H 2 /N 2 .